Prefrontal cortex reactivity underlies trait vulnerability to chronic social defeat stress Psychological stress contributes to the onset and exacerbation of nearly all neuropsychiatric disorders. Individual differences in stress-regulatory circuits can therefore dramatically affect vulnerability to these illnesses. Here we identify neural circuit mechanisms underlying individual differences in vulnerability to stress using a murine model of chronic social defeat stress. In chronically stressed mice, we find that the degree of prefrontal cortex (PFC) control of amygdala activity predicts stress susceptibility in individual mice. Critically, we also find that individual differences in PFC activation (that is, reactivity) during exposure to an aggressor mouse predict the emergence stress-induced behavioural deficits in stress-naïve mice. Finally, we show that naturally occurring differences in PFC reactivity directly correspond to the intrinsic firing rate of PFC neurons. This demonstrates that naturally occurring differences in PFC function underlie individual differences in vulnerability to stress, raising the hypothesis that PFC modulation may prevent stress-induced psychiatric disorders. Maladaptive responses to environmental stress have been implicated in the onset and exacerbation of neuropsychiatric disorders including major depressive disorder (MDD) [1] , [2] , [3] , anxiety disorder [4] , [5] , addiction [6] , [7] , schizophrenia [8] , [9] , [10] and posttraumatic stress disorder [11] . Nonetheless, individuals respond to stress differently and it remains unknown what makes some particularly vulnerable to the onset of psychiatric disorders in response to such stress. To date, studies aimed at uncovering the mechanisms underlying stress-induced behavioural dysfunction have been largely based on experiments performed in animals after exposure to stress or in animals that have been subjected to molecular, behavioural, environmental or circuit-based manipulations before stress exposure (two strategies that, in and of themselves, alter normal brain function) [12] , [13] , [14] , [15] , [16] . An alternate strategy to dissect the mechanisms that mediate trait susceptibility (that is, vulnerability to stress) is to collect data from a population of brains before exposure to stress and compare this against behaviour after stress. By identifying differences in neurophysiological signatures that can be reliably measured in stress-naïve animals, studies can be conducted to dissect the molecular and cellular mechanisms that underlie vulnerability to stress. Furthermore, these neurophysiological signatures hold great potential for use in the identification of at-risk populations and for developing therapies that promote resilience as they can be readily translated to human biomarkers. Here we use a chronic social stress model and chronic in vivo electrophysiological recordings to uncover a novel neurophysiological measure that predicts individual differences in stress tolerance in stress-naïve animals. In rodent models, chronic social defeat stress induces a behavioural syndrome characterized by social avoidance, dysfunctional reward-related behaviour and impaired coping responses to other environmental stressors [17] , [18] . Importantly, this stress-induced syndrome does not manifest in all mice within the inbred C57BL/6J (C57) strain. This behavioural variability renders the chronic social defeat stress model a powerful tool for studying the mechanisms underlying individual differences in stress resiliency and susceptibility [17] , [19] , [20] . Here we demonstrate that the response properties of PFC to AMY circuits correspond to naturally occurring differences in vulnerability to chronic social defeat stress. AMY and PFC are brain regions that are connected by reciprocal glutamatergic projections and have been shown to be important for modulating fear and stress responses. The AMY plays a critical role in detecting potential threats [21] , [22] , [23] , while the PFC executive networks provide top-down control of emotional responses by suppressing activity in the AMY [24] . Long-term stress exposure can lead to architectural changes in PFC and may alter its functional connectivity to the rest of the brain [25] . Similarly, changes in AMY activity, plasticity and gene expression following repeated stress and fear responses are profound in both humans and rodents [11] , [26] , [27] , [28] , [29] . In addition, PFC–AMY connectivity has been shown to be important in psychiatric disorders that are brought on or exacerbated by stress. Altered resting network functional connectivity between AMY and PFC has been described in patients with MDD [30] , [31] and in a genetic mouse model of MDD risk [32] . Similarly, individual differences in AMY and PFC functional connectivity following major trauma predict the manifestation of future posttraumatic stress disorder symptoms [33] . Finally, activation of the AMY in response to emotional cues correlates with trait anxiety across individuals [34] , and the structural integrity of the PFC–AMY circuit has been shown to predict trait anxiety [35] . As stress response and regulation of affect appear to be closely related to PFC–AMY connectivity, we postulate that this circuit might play a key role in mediating predisposition to the stress-induced maladaptive syndrome observed in mice after chronic social defeat stress. Here, we test our hypothesis that naturally occurring differences in PFC to AMY circuit function underlie individual differences in vulnerability to stress. To accomplish this, we recorded local field potential (LFP) and single unit activity in PFC and AMY in C57 mice before, and in response to, chronic social defeat stress. We identify several neurophysiological correlates of the susceptible phenotype in chronically stressed mice. We also demonstrate that one of these neurophysiological correlates is present across the population of stress-susceptible mice even before stress exposure (that is, neurophysiological biomarker). Finally, we quantify the changes in PFC and AMY unit firing that correspond with the manifestation of this neurophysiological profile in stress naïve mice. Together, these results demonstrate that naturally occurring difference in PFC firing rates potentially underlie individual differences in stress tolerance. Directional Signals within the PFC–AMY circuit PFC to AMY directional interactions have been described during anxiety related behaviour [36] , thus we set out to determine if PFC to AMY directional interactions occurred during our stress paradigm. C57 mice were implanted with microwire recording electrodes in PFC and AMY. Following surgical recovery, animals were subjected to 15 days of chronic social defeat stress where they were exposed to a new aggressive CD1 mouse each day and housed for 24 h adjacently with sensory contact to the CD1 (ref. 17) [17] . Neurophysiological activity was recorded during exposure to a CD1 aggressor mouse before and after chronic stress. To directly quantify neurophysiological responses to the aggressor mice, we developed a forced interaction test (FI test). During the FI test, the C57 mouse is placed in a recording chamber and neurophysiological recordings are obtained before and following introduction of a CD1 mouse into the outer arena ( Fig. 1a ). Importantly, this FI test allows for the direct quantification of circuit responses to an aggressor mouse without the influence of forward locomotor behaviours on neurophysiological measures. 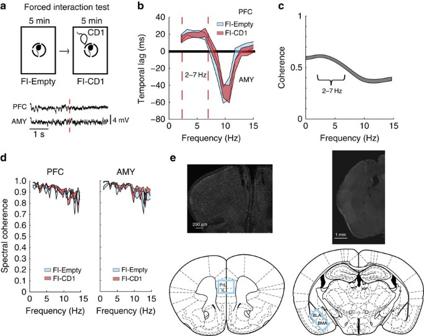Figure 1: Directional domain within the PFC–AMY circuit. (a) Schematic of the FI test performed in a 17″ × 9″ arena. PFC and AMY LFP activity recorded during post-stress FI testing. (b) The mean resultant length of the phase offset time series was calculated between the AMY and PFC LFPs. Temporal offsets where the optimal phase coherence between all AMY and PFC LFPs were observed for each frequency across 46 mice. PFC to AMY phase entrainment was observed in the 2–7 Hz oscillatory band. Data are shown as the 95% confidence interval. (c) PFC–AMY spectral coherence during the first half of the FI test. Note the high spectral coherence observed in the 2–7 Hz oscillatory band. (d) Neurophysiological activity was recorded from 16 microwires implanted in each brain area during the FI test. Intra-area spectral coherence was then calculated across implanted microwires in a mouse (N=120 unique microwire pairs for each brain area). Oscillatory signals within the 2–7 Hz range were highly redundant during the baseline and interaction periods across individual microwires implanted in a brain region (that is, coherence ~0.95). Data are shown as mean±s.e.m. (e) Individual microwires were distributed across PFC (prelimbic cortex (PrL) and infralimbic cortex (IL)) and AMY (basolateral AMY (BLA) and basomedial AMY (BMA)) throughout the anteroposterior axis. Lesion tracks are shown above. Figure 1: Directional domain within the PFC–AMY circuit. ( a ) Schematic of the FI test performed in a 17″ × 9″ arena. PFC and AMY LFP activity recorded during post-stress FI testing. ( b ) The mean resultant length of the phase offset time series was calculated between the AMY and PFC LFPs. Temporal offsets where the optimal phase coherence between all AMY and PFC LFPs were observed for each frequency across 46 mice. PFC to AMY phase entrainment was observed in the 2–7 Hz oscillatory band. Data are shown as the 95% confidence interval. ( c ) PFC–AMY spectral coherence during the first half of the FI test. Note the high spectral coherence observed in the 2–7 Hz oscillatory band. ( d ) Neurophysiological activity was recorded from 16 microwires implanted in each brain area during the FI test. Intra-area spectral coherence was then calculated across implanted microwires in a mouse ( N =120 unique microwire pairs for each brain area). Oscillatory signals within the 2–7 Hz range were highly redundant during the baseline and interaction periods across individual microwires implanted in a brain region (that is, coherence ~0.95). Data are shown as mean±s.e.m. ( e ) Individual microwires were distributed across PFC (prelimbic cortex (PrL) and infralimbic cortex (IL)) and AMY (basolateral AMY (BLA) and basomedial AMY (BMA)) throughout the anteroposterior axis. Lesion tracks are shown above. Full size image Since multiple studies have demonstrated that directional communication signals across brain circuits can be extracted from concurrently recorded LFP signals [32] , [37] , [38] , we calculated the extent to which oscillatory activity in AMY synchronized with oscillatory activity in PFC during the ‘post-stress’ FI test. We then introduced step-wise temporal offsets between PFC and AMY oscillations and recalculated the phase synchrony between these two regions. Consistent with our previous report [32] , we found that PFC activity reliably preceded AMY activity in the 2–7 Hz range across animals ( Fig. 1b ). This directionality in the coupling of PFC 2–7 Hz oscillations and AMY 2–7 Hz oscillations was observed during both periods of the FI test (that is, before and following introduction of the aggressor CD1 mouse; see Fig. 1c ; N =46 mice). Importantly, high spectral coherence was observed between PFC and AMY within this frequency band (see Fig. 1c ). High intra-area coherence was observed within animals as well, demonstrating that 2–7 Hz oscillatory signals recorded from individual microwires implanted across a given brain region were highly redundant ( Fig. 1d , see Fig. 1e for implantation sites). After identifying directional coupling between PFC and AMY LFPs, we set out to determine whether the PFC entrained AMY activity at the level of individual units. First, we quantified PFC and AMY single neuron (unit) activity in relationship to their locally recorded oscillations. Our results demonstrated that 83/236 (35%) PFC units phase locked to PFC 2–7 Hz oscillations and 37/106 (35%) AMY units phase locked to AMY 2–7 Hz oscillations (see Fig. 2a ). Exposure to the aggressor CD1 mouse decreased phase locking in the PFC phase locked units ( P <0.01 using sign-rank test; see Fig. 2b ). However, exposure to the CD1 mouse significantly increased phase locking in the population of AMY units that phase locked to AMY 2–7 Hz oscillations ( P <0.01 using sign-rank test; Fig. 2b ). Next, we calculated directionality within this circuit by introducing step-wise offsets in the PFC 2–7 Hz oscillations and calculating cross-area phase locking for AMY units. We found that AMY neurons optimally phase locked to PFC oscillations 24.6±9.2 ms in the past (N=25 neurons that exhibited significant phase locking at P <0.05/121 shifts; see Fig. 2c ). Exposure to the CD1 decreased cortical entrainment in these neurons ( Fig. 2d ; P =0.03 using sign-rank test). Notably, similar analysis using PFC units demonstrated that PFC optimally phase locked to PFC oscillations 13.9±6.4 ms in the past. This reflected an ~10 ms offset between the phase entrainment of PFC and AMY units, which is largely consistent with our LFP analysis. 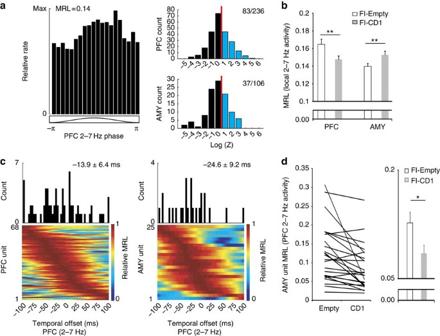Figure 2: PFC entrainment of AMY and PFC unit activity during exposure to aggressor mouse. (a) Example of unit phase locking in a PFC neuron. Data show the firing rate of a PFC neuron relative to the phase of locally recorded oscillatory activity. Significant phase locking was determined using the Rayleigh test whereZ=−ln(P). Distribution of AMY and PFC neuron phase locking values to their local 2–7 Hz oscillations are shown to the right. (b) MRL of phase-locked units shown inFig. 2a. Exposure to the aggressor mouse during ‘post-stress’ FI testing decreased the phase locking of PFC units (N=83;P<0.01) and increased the phase locking of AMY units (N=37;P<0.01). Data are shown as mean±s.e.m. (c) Mean resultant length (MRL) of PFC (left) and AMY (right) unit coupling to PFC oscillations at temporal offsets ranging from −100 to 100 ms. Only units that exhibited significant phase locking at anα=0.05/101 (−100 to 100 ms shifts in 2-ms steps) during the first half of the FI test were included in the analysis. PFC units optimally coupled to PFC oscillations 13.9±6.4 ms in the past (N=68 units). AMY units optimally coupled to PFC units 24.6±9.2 ms in the past (N=25 units). (d) Exposure to the aggressor mouse during ‘post-stress’ FI testing decreased the entrainment of AMY units to PFC oscillations. The maximum MRL for each neuron was used for analysis. *P<0.05; **P<0.01 using sign-rank test. Figure 2: PFC entrainment of AMY and PFC unit activity during exposure to aggressor mouse. ( a ) Example of unit phase locking in a PFC neuron. Data show the firing rate of a PFC neuron relative to the phase of locally recorded oscillatory activity. Significant phase locking was determined using the Rayleigh test where Z =−ln( P ). Distribution of AMY and PFC neuron phase locking values to their local 2–7 Hz oscillations are shown to the right. ( b ) MRL of phase-locked units shown in Fig. 2a . Exposure to the aggressor mouse during ‘post-stress’ FI testing decreased the phase locking of PFC units ( N =83; P <0.01) and increased the phase locking of AMY units ( N =37; P <0.01). Data are shown as mean±s.e.m. ( c ) Mean resultant length (MRL) of PFC (left) and AMY (right) unit coupling to PFC oscillations at temporal offsets ranging from −100 to 100 ms. Only units that exhibited significant phase locking at an α =0.05/101 (−100 to 100 ms shifts in 2-ms steps) during the first half of the FI test were included in the analysis. PFC units optimally coupled to PFC oscillations 13.9±6.4 ms in the past ( N =68 units). AMY units optimally coupled to PFC units 24.6±9.2 ms in the past ( N =25 units). ( d ) Exposure to the aggressor mouse during ‘post-stress’ FI testing decreased the entrainment of AMY units to PFC oscillations. The maximum MRL for each neuron was used for analysis. * P <0.05; ** P <0.01 using sign-rank test. Full size image PFC to AMY circuit function in chronically stressed mice After identifying a PFC to AMY-directed signal (that is, 2–7 Hz frequency), and characterizing the relationship of local neurons to this circuit, we set out to compare behavioural and neurophysiological responses to an aggressor mouse in chronically stressed animals. Thus, we quantified LFP responses to a CD1 aggressor mouse (using the FI test) and compared them against individual social interaction times (on a classic choice social interaction test) (see Figs 1a and 3a,b ). The interaction ratio during the choice interaction test (that is, time spent in proximal interaction to a CD1 in small chamber/time spent proximal to same empty chamber) has been validated as a strong measure of stress susceptibility or resilience [19] . Neurophysiological responses to the aggressor mouse were quantified as circuit reactivity defined as X CD1 − X Empty arena (where X represents a neurophysiological measure). We found that the change in PFC–AMY LFP coherence that resulted from the acute exposure to the aggressor negatively correlated with the interaction ratio during behavioural testing ( P =0.026, R =−0.407 using spearman rank correlation; N =30 mice; Fig. 3c ). Increases in PFC–AMY coherence were observed in mice with low social interaction ratios, while decreases in PFC–AMY coherence were observed in mice with high social interaction ratios. When we divided mice into susceptible and resilient populations based on the interaction ratio (an interaction ratio of >=0.94 corresponding with the top 40% of interaction ratios observed in the population was used to define the resilient group; N =30 total mice; interaction ratio: 1.17±0.07 for the resilient group and 0.58±0.07 for the susceptible group), we did not find differences in the change in PFC–AMY coherence between non-stressed control mice ( N =16 mice) and the susceptible or resilient groups ( P >0.05 for both comparisons using Wilcoxon rank-sum test; Fig. 3c inset). 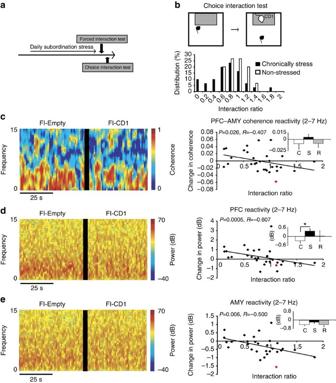Figure 3: PFC–AMY circuit dynamics correlates with stress-induced behavioral changes. (a) Schematic of experimental comparison and correlations between post-stress neurophysiological reactivity measures and post-stress social interaction behaviour. (b) Schematic of classic choice social interaction test. (c–e) PFC–AMY circuit dynamics during the post-stress FI test predicts the interaction ratio during subsequent single-chamber social interaction testing. Reactivity was quantified as the difference in each measure (that is, coherence or power) before and after the CD1 was introduced during the FI test (XCD1-Xempty arena). Data were analysed using a Spearman rank correlation (N=30 mice). Representative coherence and spectral plots for the animal highlighted in red are shown to the left. Insets show group means for non-stress control mice (C), susceptible mice (S), and resilient mice (R). *P<0.05 using FDR-corrected rank-sum test. Data are shown as mean±s.e.m. Figure 3: PFC–AMY circuit dynamics correlates with stress-induced behavioral changes. ( a ) Schematic of experimental comparison and correlations between post-stress neurophysiological reactivity measures and post-stress social interaction behaviour. ( b ) Schematic of classic choice social interaction test. ( c – e ) PFC–AMY circuit dynamics during the post-stress FI test predicts the interaction ratio during subsequent single-chamber social interaction testing. Reactivity was quantified as the difference in each measure (that is, coherence or power) before and after the CD1 was introduced during the FI test ( X CD1 - X empty arena ). Data were analysed using a Spearman rank correlation ( N =30 mice). Representative coherence and spectral plots for the animal highlighted in red are shown to the left. Insets show group means for non-stress control mice (C), susceptible mice (S), and resilient mice (R). * P <0.05 using FDR-corrected rank-sum test. Data are shown as mean±s.e.m. Full size image Given this interesting correlation of the PFC–AMY oscillatory coherence with social interaction, we next evaluated changes in oscillatory power (i.e., reactivity) within the 2–7 Hz band in each brain region individually (PFC and AMY). Both PFC and AMY power reactivity negatively correlated with the behavioural responses of individual C57 animals during the choice interaction test ( P =0.0005, R =−0.607 and 0.006, R =−0.500 for both comparisons, respectively, using spearman rank correlation; see Fig. 3d,e ). When we compared these neurophysiological responses in stress-susceptible and stress-resilient mice with non-stressed controls, we found that stress-susceptible mice exhibited an increase in PFC reactivity ( P <0.004 using Wilcoxon rank-sum test; Fig. 3d inset). Neither group exhibited differences in AMY reactivity compared with non-stressed controls ( P >0.05 using Wilcoxon rank-sum test; Fig. 3e inset). Correlates of vulnerability in stress-naïve mice After identifying neurophysiological correlates of stress susceptibility and resilience in chronically stressed mice (that is, PFC–AMY 2–7 Hz reactivity, PFC 2–7 Hz reactivity and AMY 2–7 Hz reactivity), we hypothesized that there might be ‘neural signature’ present in the same population of mice before chronic stress exposure. The existence of such a signature would be of enormous benefit to studying the causes of stress susceptibility, as it would enable the identification of susceptible animals in a pre-stressed state (that is, before the emergence of behavioural symptoms). Thus, we compared neurophysiological responses measured during an FI test session performed before chronic stress exposure with behavioural responses measured during post-stress choice interaction testing ( Fig. 4 , top left). Interestingly, we found that the change in PFC 2–7 Hz oscillatory power during FI testing in stress-naïve mice correlated with the degree of individual susceptibility observed across the same cohort of mice after chronic social defeat stress ( P =0.005, R =−0.508 using spearman rank correlation; Fig. 4 ). Importantly, in non-stressed control mice, no relationship was observed between PFC 2–7 Hz reactivity in chronic stress-naïve mice and ‘post-stress’ interaction scores ( P =0.831 using spearman rank correlation; N =16 mice), demonstrating that a circuit (PFC reactivity) × environment (stress) interaction was required to induce the behavioural changes observed in stress-susceptible mice. Neither PFC–AMY coherence nor AMY power reactivity (2–7 Hz) in chronic stress-naïve mice was predictive of post-stress social interaction behaviour. 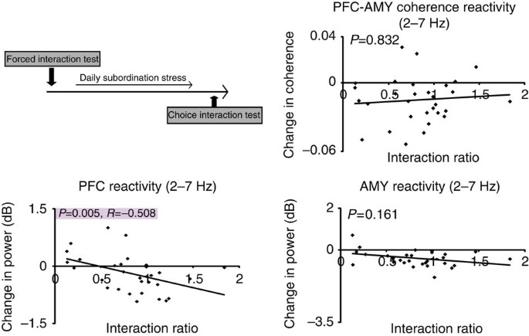Figure 4: PFC reactivity in stress-naïve mice predicts susceptibility to chronic stress. Schematic of experimental comparison and correlations between pre-stress neurophysiological reactivity measures and post-stress social interaction behaviour (data were analysed using Spearman rank correlation;N=30 mice). Figure 4: PFC reactivity in stress-naïve mice predicts susceptibility to chronic stress. Schematic of experimental comparison and correlations between pre-stress neurophysiological reactivity measures and post-stress social interaction behaviour (data were analysed using Spearman rank correlation; N =30 mice). Full size image PFC and AMY neuronal activity profiles in stress-naïve mice Since our evidence demonstrated that PFC power reactivity in the 2–7 Hz band was a neurophysiological correlate of trait vulnerability to stress, we set out to investigate if this neurophysiological marker was sufficient to segregate stress-naïve mice and probe the cellular mechanisms that may underlie trait vulnerability to stress. To increase the number of neurons used for analysis, we used all pre-stress FI test data recorded in mice that would later be subjected to chronic social defeat stress or assigned to serve as non-stressed controls. We then divided mice into two groups based on their PFC power reactivity (high PFC reactivity: HPR; PFC reactivity >−0.37 dB, N =25/51 mice. Low PFC reactivity: LPR; PFC reactivity <−0.37 dB, N =26/51 mice), and compared unit responses during the pre-stress FI test in these two groups. We found that LPR mice display higher PFC firing rates compared with the HPR group during both portions of the FIT (mixed model analysis of variance with Box–Cox transformation (MMA) of reactivity group; F 1,296 =6.8039, P =0.0096; N =127 and 171 PFC neurons in HPR and LPR mice respectively; Fig. 5a ). In addition, PFC firing rates increase during exposure to the CD1 aggressor mouse in LPR, but not HPR mice (MMA of test condition; F 1,296 =14.732, P =0.0002; followed by false discovery rate (FDR)-corrected Wilcoxon sign-rank test (MMA–FWS); P =0.0014 and 0.06 for LPR and HPR mice, respectively). No group differences in AMY firing rates were observed between LPR and HPR mice (MMA of reactivity group; F 1,152 =0.012, P =0.913; N =62 and 92 AMY neurons in HPR and LPR mice, respectively; Fig. 5a ). Similarly, no group differences in unit phase locking to PFC 2–7 Hz oscillations were observed in AMY (MMA of reactivity group; F 1,114 =2.60, P =0.110; N =49 and 67 AMY neurons in HPR and LPR mice, respectively) or PFC (MMA of reactivity group; F 1,114 =2.18, P =0.141; N =112 and 163 PFC neurons in HPR and LPR mice, respectively; Fig. 5a ). Finally, we compared cortical and AMY phase locking to AMY 2–7 Hz oscillations in the two groups. We found that HPR mice displayed higher AMY phase locking to AMY 2–7 Hz oscillations (MMA of reactivity group; F 1,114 =6.35, P =0.0132; N =49 and 67 AMY neurons in HPR and LPR mice, respectively; Fig. 5a ). LPR mice tended to exhibit higher PFC unit phase locking to AMY oscillations, although these differences did not reach statistical significance (MMA of reactivity group × test condition; F 1,273 =6.41, P =0.012; followed by FDR-corrected rank-sum test; P =0.064 for comparisons between groups within the first half of the FI test; Fig. 5a ). Exposure to the aggressor mouse decreased PFC unit phase locking to AMY oscillations in the LPR, but not HPR group ( P =0.004 and 0.754 for comparisons within the LPR and HPR group during the FI test using FDR-corrected Wilcoxon sign-rank test; Fig. 5a ). Taken together, these results demonstrate that LPR mice exhibit higher PFC firing rates and lower AMY coupling to local AMY oscillatory activity. Importantly, these results also provide evidence that PFC reactivity can indeed be used as a neurophysiological marker to segregate stress-naïve mice and probe the cellular mechanisms underlying trait vulnerability to stress. 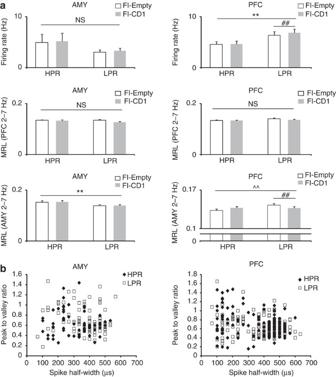Figure 5: Unit activity profiles corresponding with PFC reactivity. (a) Unit activity profiles in stress-naïve mice during pre-stress FI testing. Mice were segregated into two groups based on their naturally occurring differences in PFC spectral reactivity (N=25–26 mice per group). Data are shown as mean±s.e.m. **P<0.01 for reactivity group effect using MMA of reactivity group × test condition with Box–Cox transform; ^^P<0.01 for MMA of reactivity group × test condition interaction.##P<0.01 for test condition effect using sign-rank test. (b) Units waveform properties. Note the overlapping distribution of waveform properties in LPR and HPR mice. Figure 5: Unit activity profiles corresponding with PFC reactivity. ( a ) Unit activity profiles in stress-naïve mice during pre-stress FI testing. Mice were segregated into two groups based on their naturally occurring differences in PFC spectral reactivity ( N =25–26 mice per group). Data are shown as mean±s.e.m. ** P <0.01 for reactivity group effect using MMA of reactivity group × test condition with Box–Cox transform; ^^ P <0.01 for MMA of reactivity group × test condition interaction. ## P <0.01 for test condition effect using sign-rank test. ( b ) Units waveform properties. Note the overlapping distribution of waveform properties in LPR and HPR mice. Full size image Chronic social defeat stress in rodents induces a behavioural syndrome characterized by social avoidance and impaired coping responses to other environmental stressors in susceptible individuals that parallels stress-induced affective dysfunction in humans. Within the inbred (genetically identical) C57 mouse strain, this stress-induced phenotype does not occur in all animals, allowing for dissection of the factors that mediate susceptibility and resilience to stress [17] , [19] , [20] . Identifying the underlying differences inherent in the brain circuitry of susceptible and resilient animals before exposure to chronic social stress opens the door for the development of novel therapies and prevention strategies that enable stress resistance. Both the PFC and AMY have been shown to play important roles in stress-related syndromes in humans and in rodents [21] , [22] , [23] , [30] , [31] , [32] , [33] , [36] , [39] , [40] . Here, we characterized the activity of the PFC–AMY circuit in C57 mice with respect to chronic social defeat stress. Our results demonstrated that functional changes in PFC–AMY coherence, PFC oscillatory activity and AMY oscillatory activity in response to exposure to an aggressor mouse correlated with individual differences in behavioural responses to a similar aggressor mouse in chronically stressed mice. Importantly, these relationships were observed across the 2–7 Hz frequency band that reflects PFC to AMY-directed activity. Thus, the PFC–AMY circuit reactivity observed here may reflect the activation of a feedback regulatory network that suppresses subcortical neurophysiological responses to stressful stimuli. This feedback control network appears to work more efficiently in the resilient animals, which have greater suppression of AMY oscillatory activity in response to the aggressor CD1. In stress-susceptible mice, downstream de-potentiation of this regulatory network in response to chronic stress may result in a compensatory upregulation in the PFC-mediated response. Indeed, higher PFC reactivity was observed in stress-susceptible (but not resilient) mice, compared with non-stressed controls. We also show that PFC power reactivity in stress-naïve mice correlates with the behavioural changes that emerge following chronic stress. Notably, both PFC–AMY coherence and AMY oscillatory power reactivity in stress-naïve mice failed to predict post-stress behavioural responses. This is likely because the chronic stress is required to unmask downstream circuit-level deficits in the feedback regulatory networks of vulnerable animals. When we explored individual differences in firing at the level of cellular ‘units’, we found that LPR (a predictor of low vulnerability to chronic stress) was associated with higher PFC firing rates, and lower AMY coupling to local 2–7 Hz oscillatory activity. Previous studies have suggested that PFC outputs to downstream limbic targets mediate the effects of behavioural manipulations that enhance resilience to chronic social defeat stress [16] . Furthermore, direct stimulation of PFC is sufficient to reverse several of the behavioural deficits that emerge following chronic stress exposure [14] , [15] , [41] . Taken together with our findings, this suggests that the increased PFC activity observed in the LPR mice likely serves to suppress stress responses in subcortical brain regions thereby increasing tolerance to chronic stress. Anatomical subdivisions of PFC, including prelimbic (PrL) cortex and infralimbic (IL) cortex, have been shown to play diverse and divergent roles in mediating responses to fearful stimuli [42] . While individual microwires were distributed across these two subdivisions of PFC in our study, we found high intra-PFC coherence within the 2–7 Hz range. The predictive neural responses we observed in PFC may reflect the integration of activity across several PFC nodes that ultimately contribute to long-term responses to stress. Alternatively, the high intra-area coherence observed across the PFC in the 2–7 Hz frequency range may simply reflect the result from the local volume conduction of LFP signals [43] . Additional studies would aid in dissecting the contribution of individual LFP nodes to the PFC 2–7 Hz regulatory network. Multiple subcortical neural circuits play a role in mediating behavioural responses to stress and the behavioural changes that occur in response to chronic stress. Indeed, dopamine-dependent brain circuit adaptations in VTA have been shown to contribute to the emergence of the severe behavioural disturbances displayed by stress-susceptible mice after stress exposure [12] , [13] , [19] , [44] , [45] , and changes in these dopamine-dependent circuits have also been shown to accompany the reversal of behavioural symptoms following antidepressant administration [44] . Nevertheless, differences in dopaminergic-dependent circuits that exist before stress exposure and ultimately mediate the individual differences in stress tolerance observed within the C57 mouse strain have not been identified. Our findings demonstrate that naturally occurring differences in PFC activity likely serve as a trait phenotype of stress susceptibility and resilience. Since activation of PFC-dependent circuits is sufficient to regulate activity in multiple subcortical targets [15] , our findings also raise the hypothesis that the PFC may regulate the dopamine-dependent encoding of stress responses, and that naturally occurring differences in PFC firing activity may result in vulnerability to stress in several downstream circuits. Our findings provide the first direct evidence, to our knowledge, that the PFC–AMY circuit encodes the individual capacity to maintain normal behaviour in the face of severe stress. Importantly, we describe a novel neurophysiological marker that can be used to quantify susceptibility in intact stress-naïve mice. This neurophysiological marker can be assessed at the level of LFPs allowing for reliable and rapid high-throughput classification of animals into stress-vulnerable and stress-tolerant populations. Thus, use of such a neurophysiological biomarker enables a deeper investigation into the molecular- and cellular-based brain mechanisms that ultimately determine individual stress vulnerabilities. Animal care and use C57BL/6J (C57) male mice purchased from the Jackson Labs and CD1 male mice (retired breeders) purchased from Charles River Laboratory were used for all experiments presented in this study. Mice were housed on a reversed 12-h light/dark cycle, and maintained in a humidity- and temperature-controlled room with water and food available ad libitum . C57 mice were initially housed three–five per cage and CD1 mice were singly housed. Behavioural and electrophysiological experiments were conducted during the dark cycle. All studies were conducted with approved protocols from the Duke University Institutional Animal Care and Use Committee and were in accordance with the NIH guidelines for the Care and Use of Laboratory Animals. Electrode implantation surgery At an age of 6–7 weeks, 51 C57 mice ( N =51) were separated into individual cages. C57 mice were anesthetized with ketamine (100 mg kg −1 ) and xylazine (10 mg kg −1 ), placed in a stereotaxic device and metal ground screws were secured to the cranium. A total of 32 tungsten microwires were arranged in array bundles and implanted in AMY and PFC based on stereotaxic coordinates measured from bregma (AMY: −1.6 mm anteroposterior, −2.5 mm mediolateral, −4.8 mm dorsoventral from the dura; PFC: 1.7 mm anteroposterior, ±0.25 mm mediolateral, −1.8 to −2.5 mm dorsoventral from the dura). Implanted electrodes were anchored to ground screws above anterior cranium and cerebellum using dental acrylic [46] . Experiments were initiated following a 2-week recovery. Histological analysis of implantation sites was performed at the conclusion of experiments. Chronic social defeat stress Experimental mice underwent 15 days of chronic social defeat stress [17] , [41] . Male, retired breeder CD1 (Charles River) mice were used as resident aggressors for the social defeat stress and were singly housed before the experiments. Particularly aggressive CD1s, as defined by demonstrating at least one successful act of aggression towards an intruder C57 male within 60 s, were selected for use during the social defeat. Mice were singly housed before undergoing social defeat. Intruder male C57 mice were introduced to the cage of a novel CD1 aggressor for 5 min daily, and then housed adjacent to the same aggressor for 24 h. During this time, mice were separated by a transparent and porous Plexiglas barrier to enable constant sensory exposure. During bouts of exposure to the CD1 mice, hallmark behavioural signs of social defeat stress were observed including escape, submissive postures (that is, defensive upright and supine), and freezing. Following the last 24 h exposure to a CD1 aggressor mouse, all C57s were housed individually. Non-stressed control animals were housed in identical cages adjacent to another C57 of the same age on the opposite side of Plexiglas barrier and handled each day. FI test C57 mice were placed in a wire cage (Galaxy Utility Cup, www.kitchen-plus.com ) in the middle chamber of a 17 × 9 × 9 (L × W × H inch) arena. The dimensions of the wire cage were 4 × 4 × 3″ (lower diameter × height × upper diameter). Following a 5-minute recording period during which neurophysiological activity was recorded, a CD1 aggressor mouse was introduced into the center chamber. Neurophysiological data were then recorded for an additional 5 minutes. All animals subjected to the FI test after exposure to chronic social defeat stress were also subjected to the test before stress exposure. Mice that exhibited significant injuries during social defeat stress were removed from further post-stress testing ( N =5 mice). Single-chamber social interaction test Mice were subjected to the single-chamber social interaction test following chronic social defeat stress. Mice were placed within a novel arena with a small cage located at one end, and each socially stressed mouse’s movement was monitored for 2.5 min. Mice were then removed from the testing chamber, and reintroduced 30 s later after a CD1 mouse was placed in the small cage along. Locomotor activity measurements (distance travelled) and time spent in the interaction zone were quantified using Ethovision 3.0 software. The interaction ratio was calculated as (interaction time, CD1 present)/(interaction time, CD1 absent). Data were analysed using a Student’s t -test at α =0.05. Neurophysiological data acquisition Neurophysiological recordings were performed during the FI test. Neuronal activity was sampled at 30 kHz, high-pass filtered at 250 Hz, sorted online and stored using the Cerebus acquisition system (Blackrock Microsystems, UT). Neuronal data were referenced online against a wire within the same brain area that did not exhibit a signal-to-noise ratio greater than 3:1. At the end of the recording, cells were sorted again using an offline sorting algorithm (Plexon, TX) to confirm the quality of the recorded cells. LFPs were band-pass filtered at 0.3–500 Hz and stored at 1,000 Hz. All neurophysiological recordings were referenced to a ground wire connected to both ground screws. Notably, wires tested from the two screws were isoelectric demonstrating that ground loops were not introduced by this design. LFP oscillatory power and cross-area coherence Signals recorded from all of the implanted microwires were used for analysis. High intra-area coherence was observed within animals (see Fig. 1d ), demonstrating that oscillatory signals recorded from individual microwires implanted across a given brain region were highly redundant (particularly in the frequency range examined in this study) [43] . Using Matlab, a sliding window Fourier transform was applied to the LFP signal using a 1-s window with a 1-s step. The Fourier transform parameters were then chosen to allow for a frequency resolution of 0.5 Hz. The LFP oscillatory power values used for analysis were then assigned as the mean power observed across the two LFP channels used for analysis. LFP cross-structural coherence was then calculated from LFP pairs used for LFP oscillatory power analysis using the Matlab (MathWorks, Natick, MA) mscohere function at a 1-s sliding window with a 1-s step. The transform parameters were chosen to allow for a frequency resolution of 0.5 Hz. The average of the calculated coherence value across all wires was used for analysis. Unit phase locking LFPs were filtered using Butterworth band-pass filters designed to isolate LFP oscillations within the delta (2–7 Hz) frequency range. The instantaneous phase of the filtered LFP was then determined using the Hilbert transform, and phase locking was detected using the Rayleigh test at α =0.05 (refs 47 , 48 ). Since the phase-locking analysis is highly influenced by the number of spike events used for analysis, we quantified the strength of unit phase locking by randomly selecting exactly fifty spike events for each neuron and calculating the MRL. This process was repeated 1,000 times for each neuron and the average MRL observed across the 1,000 samples was used to quantify phase locking for each neuron [49] . Neurons that fired fewer than 50 times were excluded from phase-locking analysis. All behavioural state comparisons of phase locking were performed using the MRL of neurons. Temporal offset for optimal phase coupling First, we calculated the cross-correlation of instantaneous phases of field potential oscillations to determine the temporal lag that yielded the correlation peak. This was then used as an indication of directionality. Similar approaches based on instantaneous amplitude correlations have been described in the literature [37] . Briefly, LFP data acquired during the first 5 min of each recording period were filtered using Butterworth band-pass filters designed to isolate LFP oscillations within a 2 Hz window using a 1 Hz step (2–15 Hz). The instantaneous phase of the filtered AMY and PFC LFPs were then determined using the Hilbert transform, and the instantaneous phase offset ( φ AMY− φ PFC ) t was calculated for each time point. The mean resultant length for the phase offset time series, corresponding to the deviation from circular uniformity (where 0 represents no deviation from circular uniformity and 1 represents a perfect distribution at a single angle/phase) was then calculated [32] . Second, we introduced temporal shifts ranging from −100 to 100 ms in 2-ms increments into PFC oscillations. We then recalculated the MRL length of coupling between the temporally shifted PFC oscillations and the population of PFC and AMY neurons we recorded. This approach has been previously utilized to quantify directionality across limbic neural circuits [36] . All neurophysiological and behavioural tests were completed before data analysis. All data in the text are presented as mean±s.e.m unless otherwise specified. How to cite this article : Kumar, S. et al. Prefrontal cortex reactivity underlies trait vulnerability to chronic social defeat stress. Nat. Commun. 5:4537 doi: 10.1038/ncomms5537 (2014).